Association between Gαi2 and ELMO1/Dock180 connects chemokine signalling with Rac activation and metastasis The chemokine CXCL12 and its G-protein-coupled receptor CXCR4 control the migration, invasiveness and metastasis of breast cancer cells. Binding of CXCL12 to CXCR4 triggers activation of heterotrimeric Gi proteins that regulate actin polymerization and migration. However, the pathways linking chemokine G-protein-coupled receptor/Gi signalling to actin polymerization and cancer cell migration are not known. Here we show that CXCL12 stimulation promotes interaction between Gαi2 and ELMO1. Gi signalling and ELMO1 are both required for CXCL12-mediated actin polymerization, migration and invasion of breast cancer cells. CXCL12 triggers a Gαi2-dependent membrane translocation of ELMO1, which associates with Dock180 to activate small G-proteins Rac1 and Rac2. In vivo , ELMO1 expression is associated with lymph node and distant metastasis, and knocking down ELMO1 impairs metastasis to the lung. Our findings indicate that a chemokine-controlled pathway, consisting of Gαi2, ELMO1/Dock180, Rac1 and Rac2, regulates the actin cytoskeleton during breast cancer metastasis. Metastasis is the transmission of cancerous cells from an original site to other selective organs elsewhere in the body. In breast cancer patients, secondary tumours are often found in the lungs, lymph nodes and bone marrow [1] , [2] . Previous studies have shown that chemokine-mediated cancer cell migration, chemotaxis, determines the specificity of metastasis to target organs [1] , [2] , [3] . Chemokines are small proteins that function as extracellular signals detected by a subfamily of G-protein-coupled receptors (GPCRs). Chemokines and their receptors normally guide leukocytes to sites of infection and inflammation, and also control the trafficking of lymphocytes [4] . Cancer cell migration shares similarities with leukocyte migration. For example, in a mouse model, the chemokine CXCL12 (also known as SDF-1α) and its receptor CXCR4 control the metastasis of breast cancer cells to lung and bone marrow, where expression of CXCL12, a ligand of CXCR4 on breast cancer cells, is high [1] , [2] , [5] . Alteration of the expression pattern of chemokine receptors on the breast cancer cell surface changes the metastasis target organs, and inhibition of chemokine receptors blocks metastasis [1] , [4] , [5] . However, it is not known how chemokines and their receptors regulate the actin cytoskeleton leading to metastasis of cancer cells. Thus, it is of critical importance to study chemokine receptor-mediated signalling pathways in breast cancer cells. Activation of a chemokine receptor promotes the dissociation of the heterotrimeric G-proteins, Gαi and Gβγ, which in turn activates downstream signal transduction pathways that ultimately regulate the spatiotemporal organization of the actin cytoskeleton to drive cell migration [6] , [7] , [8] , [9] , [10] . In leukocytes, chemokine receptors control activation of a small G-protein, Rac, which induces growth of actin filaments by removing capping proteins and by stimulating the Arp2/3 complexes that initiate the formation of new actin branches from existing ones [7] , [11] . The extension of the dendritic actin cytoskeleton drives the membrane forward, resulting in cell migration [12] , [13] . Activation of Rac requires guanine nucleotide exchange factors (GEFs) [6] , [7] . ELMO/Dock180 complexes are evolutionarily conserved and serve as GEFs for Rac proteins controlling actin cytoskeleton in Dictyostelium discoideum , Caenorhabditis elegans , mouse and human [14] , [15] , [16] , [17] . Upon activation of an ELMO/Dock180 complex, the Dock180 protein exposes its Docker domain, which in turn binds to and activates Rac [6] , [14] , [18] . It has been shown that RhoG, a small G-protein, interacts with ELMO and controls ELMO/Dock180 to activate Rac1 during neurite outgrowth induced by nerve growth factor [19] or during phagocytosis of apoptotic cells in C. elegans [20] . A previous report has indicated that the ELMO1/Dock180 complex serving as a GEF for Rac1 has an important role in promoting cancer cell invasion [21] . A recent study in D. discoideum , a simple model organism, has shown that activation of a GPCR promotes an interaction between heterotrimeric G-protein βγ subunits and the ELMO/Dock complex, which controls chemotaxis [1] , [16] . Despite extensive studies, we still do not know how a chemokine GPCR regulates the functions of ELMO/Dock180 complexes in mammalian cells. In addition, we do not know whether the ELMO/Dock180 complex has a role in CXCL12-mediated metastasis of breast cancer cells. Here we demonstrate that ELMO1 associates with Gαi2 and interacts with Dock180 to activate Rac proteins, thereby contributing to actin polymerization in breast cancer cells. Our study reveals a novel pathway, consisting of Gαi2, ELMO1/Dock180 and Rac1/2, which has an important role in CXCL12-mediated chemotaxis and metastasis of breast cancer cells. ELMO1 functions in breast cancer chemotaxis and invasion To determine which ELMO proteins were involved in the migration of breast cancer cells, we first examined the expression of ELMOs in various breast cancer cells. Expression of ELMO1 and ELMO2 was examined in nine human cell lines, including MDA-MB-231, BT549, ZR-75-30, T47D, MCF-7, Bcap-37, SKBR3, MCF10A and HBL100, by western blotting analyses ( Fig. 1a ). Our result indicated that ELMO1 and ELMO2 were expressed in these nine cell lines, and protein levels of ELMO1 and ELMO2 were relatively high in metastatic breast cancer cells, such as MDA-MB-231 and BT549. 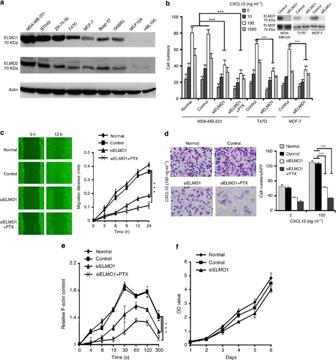Figure 1: ELMO1 functions in breast cancer chemotaxis and invasion. (a) Western blotting analysis of ELMOs endogenous expression in MDA-MB-231, BT549, ZR-75-30, T47D, MCF-7, Bcap-37, SKBR3, MCF10A and HBL100 cells. Actin was used as control. (b) Chemotaxis analysis of ELMO1 knockdown cells. Western blotting analysis of ELMO1 expression in MDA-MB-231, T47D and MCF-7 breast cancer cells. ELMO2 was used as a loading control (points=mean of three independent experiments; scale bars=s.e.m.;n=6; two-way analysis of variance (ANOVA), ***P<0.0001). (c) Scratch assay of siELMO1 cells. MDA-MB-231 cells were plated in six-well plates and formed a fluent monolayer. The medium was replaced by a RPMI medium supplied with 1% BSA. One of ELMO1 siRNA wells was pretreated with 0.1 μg ml−1PTX in medium for 2 h. The gap distance was measured at 0, 3, 6, 9, 12 and 24 h (points=mean of three independent experiments; scale bars=s.e.m.;n=6; two-way ANOVA, ***P<0.0001). (d) The reduction of ELMO1 impaired invasion of MDA-MB-231 cells, especially under 0.1 μg ml−1PTX treatment for transfected ELMO1 siRNA cells (points=mean of three independent experiments; scale bars=s.e.m.;n=6; two-way ANOVA, ***P<0.0001). (e) Actin polymerization in siELMO1 cells was decreased. Time course of relative F-actin content in normal, control, siELMO1 and siELMO1+0.1 μg ml−1PTX cells followed by CXCL12 stimulation. The value was measured at 0, 4, 8, 15, 30, 60, 120 and 300 s (points=mean of three independent experiments; scale bars=s.e.m.;n=6; two-way ANOVA, ***P<0.0001). (f) MTT assay: cell proliferation activity was not inhibited in siELMO1 cells (points=mean of three independent experiments; scale bars=s.e.m.;n=6; one-way ANOVA,P=0.8725>0.05). Figure 1: ELMO1 functions in breast cancer chemotaxis and invasion. ( a ) Western blotting analysis of ELMOs endogenous expression in MDA-MB-231, BT549, ZR-75-30, T47D, MCF-7, Bcap-37, SKBR3, MCF10A and HBL100 cells. Actin was used as control. ( b ) Chemotaxis analysis of ELMO1 knockdown cells. Western blotting analysis of ELMO1 expression in MDA-MB-231, T47D and MCF-7 breast cancer cells. ELMO2 was used as a loading control (points=mean of three independent experiments; scale bars=s.e.m. ; n =6; two-way analysis of variance (ANOVA), *** P <0.0001). ( c ) Scratch assay of siELMO1 cells. MDA-MB-231 cells were plated in six-well plates and formed a fluent monolayer. The medium was replaced by a RPMI medium supplied with 1% BSA. One of ELMO1 siRNA wells was pretreated with 0.1 μg ml −1 PTX in medium for 2 h. The gap distance was measured at 0, 3, 6, 9, 12 and 24 h (points=mean of three independent experiments; scale bars=s.e.m. ; n =6; two-way ANOVA, *** P <0.0001). ( d ) The reduction of ELMO1 impaired invasion of MDA-MB-231 cells, especially under 0.1 μg ml −1 PTX treatment for transfected ELMO1 siRNA cells (points=mean of three independent experiments; scale bars=s.e.m. ; n =6; two-way ANOVA, *** P <0.0001). ( e ) Actin polymerization in siELMO1 cells was decreased. Time course of relative F-actin content in normal, control, siELMO1 and siELMO1+0.1 μg ml −1 PTX cells followed by CXCL12 stimulation. The value was measured at 0, 4, 8, 15, 30, 60, 120 and 300 s (points=mean of three independent experiments; scale bars=s.e.m. ; n =6; two-way ANOVA, *** P <0.0001). ( f ) MTT assay: cell proliferation activity was not inhibited in siELMO1 cells (points=mean of three independent experiments; scale bars=s.e.m. ; n =6; one-way ANOVA, P =0.8725>0.05). Full size image CXCL12-mediated migration and invasion of breast cancer cells is essential for metastasis of breast cancer [1] . To study the role of ELMOs in the migration of human breast cancer cells, we specifically downregulated ELMO1 expression in a human breast carcinoma cell line, MDA-MB-231, and two other breast cancer cell lines, T47D and MCF-7, using a small interference RNA (siRNA) method (siELMO1 for ELMO1 knockdown and control for cells transfected with siRNA vector containing a scrambled insert; Fig. 1b ). Using an in vitro transwell assay, we found that CXCL12 clearly induced chemotaxis of MDA-MB-231, T47D and MCF-7 cells, whereas knockdown of ELMO1 inhibited CXCL12-induced chemotaxis in each of the three cell lines ( Fig. 1b ). A scratch assay indicated that siELMO1 cells were defective in migration ( Fig. 1c ). To test CXCL12-mediated invasion of MDA-MB-231 cells, we used an in vitro matrigel assay ( Fig. 1d ). MDA-MB-231 cells (normal and control) displayed a clear invasion, whereas siELMO1 cells were defective in CXCL12-mediated invasion. A treatment of the pertussis toxin (PTX), which is a specific inhibitor of Gαi and blocks Gαi signalling to its downstream components, further inhibited chemotaxis ( Fig. 1b ) and migration ( Fig. 1c ), and completely blocked CXCL12-mediated invasion of MDA-MB-231 cells ( Fig. 1d ). Chemokine binding to receptors triggers intracellular actin polymerization in breast cancer cells, which is essential for breast cancer cell migration and invasion. Consistent with previous studies, CXCL12 induced a transient increase (about 1.8-fold) in intracellular F-actin level in MDA-MB-231 cells within 30 s ( Fig. 1e ), whereas the CXCL12-induced actin polymerization was decreased in siELMO1 cells and reduced even more when cells were treated with PTX ( Fig. 1e ). We also examined the role of ELMO1 in the proliferation of MDA-MB-231 using an MTT (3-(4,5-dimethylthiazol-2-yl)-2,5-diphenyltetrazolium bromide) assay ( Fig. 1f ) and found that siELMO1 cells exhibited no significant reduction of cell proliferation. In addition, we found that ELMO1 was not required for cell migration and actin polymerization mediated by epidermal growth factor (EGF) and its receptor (a tyrosine kinase receptor; Supplementary Fig. S1B,C), suggesting that ELMO1 was involved in chemokine GPCR-, but not EGF receptor-, mediated chemotactic responses. Taken together, our results indicated that ELMO1 was not required for cell division, but was involved in CXCL12-mediated and Gαi-controlled migration and invasion of breast cancer cells. Amino-terminal portion of ELMO1 interacts with Gαi2 subunit To reveal the potential molecular mechanism of ELMO1 function, we sought to identify proteins that associated with ELMO1. ELMO1-YFP, expressed in CXCL12-stimulated MDA-MB-231 cells, was partially purified from lysates by using anti-green fluorescent protein (GFP) antibodies coupled to beads, and elutes were subjected to SDS gel electrophoresis. The YFP protein expressed in the cells was used as a control ( Fig. 2a ). Three prominent protein bands, which appeared in the ELMO1-YFP, but not in the control sample, were identified using mass spectrometry ( Fig. 2a and Table 1 ). The identified proteins were ELMO1-YFP, Dock180 and Gαi2 ( Table 1 ). It is well known that Dock180 and ELMO1 form a complex that serves as a GEF for small G-protein Rac to mediate actin polymerization for cell migration [17] , and Gαi2 is a subunit of heterotrimeric G-proteins that link to chemokine receptors [22] , [23] . The associations between ELMO1/Dock180 and ELMO1/Gαi2 were confirmed by immunoprecipitation analyses ( Fig. 2b ). In pulldowns of lysates from cells expressing ELMO1-YFP using an anti-GFP antibody, we found that Dock180 coimmunoprecipitated with ELMO1-YFP but not the YFP control. Similar levels of Dock180 were pulled down from the cells with or without CXCL12 stimulation or PTX treatment, suggesting that ELMO1 and Dock180 formed a stable complex, which was independent of the activation of CXCR4 receptor or heterotrimeric G-proteins. Gαi2 was also coimmunoprecipitated with ELMO1-YFP but not with YFP (control). When the cells were treated with CXCL12 and GTPγS, which activates heterotrimeric G-proteins, the association was increased, whereas the association was clearly decreased upon PTX treatment ( Fig. 2b ), suggesting that activation of CXCR4 and heterotirmeric G-proteins promoted the association between Gαi2 and the complex of ELMO1 and Dock180. 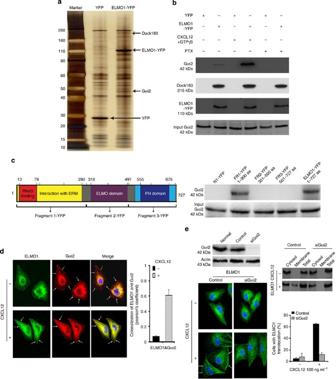Figure 2: N-terminal portion of ELMO1 interacts with Gαi2 subunit. (a) Image of SDS–PAGE gel stained by silver stain. Lysates of MDA-MB-231 cells expressing ELMO1-YFP or YFP (as a control) were incubated with beads coupled with anti-GFP antibodies and stained with silver stain. (b) Coimmunoprecipitation assay of ELMO1-YFP, Gαi2 and Dock180. The immunoprecipitation was performed by using the μMACS GFP isolation kit. The eluted proteins were separated by SDS–PAGE and were probed with antibodies. Input Gαi2 was used as control. (c) N terminus of ELMO1 was required for the interaction with Gαi2. YFP served as a negative control and ELMO1-YFP was a positive control. (d) CXCL12-induced ELMO1 colocalization with Gαi2 on the plasma membrane by confocal microscopy analysis. After stimulation with 100 ng ml−1CXCL12 for 1 h at 37 °C, cells were fixed, permeabilized and blocked in 3% BSA. MDA-MB-231 cells were stained with anti-ELMO1, anti-Gαi2 antibodies and probed with an Alexa Fluor 488-conjugated or 546-conjugated secondary antibody. Colocalization efficiency was calculated through Image J software. (e) Knockdown of Gαi2 impaired CXCL12-induced membrane translocation of ELMO1. After stimulation with 100 ng ml−1CXCL12 for 1 h at 37 °C, cells were fixed, permeabilized and blocked in 3% BSA. Twenty-five images were analysed by ImageJ software. Western blotting analysis of biochemical fractionation showed a clear enrichment of ELMO1 upon CXCL12 stimulation. Figure 2: N-terminal portion of ELMO1 interacts with Gαi2 subunit. ( a ) Image of SDS–PAGE gel stained by silver stain. Lysates of MDA-MB-231 cells expressing ELMO1-YFP or YFP (as a control) were incubated with beads coupled with anti-GFP antibodies and stained with silver stain. ( b ) Coimmunoprecipitation assay of ELMO1-YFP, Gαi2 and Dock180. The immunoprecipitation was performed by using the μMACS GFP isolation kit. The eluted proteins were separated by SDS–PAGE and were probed with antibodies. Input Gαi2 was used as control. ( c ) N terminus of ELMO1 was required for the interaction with Gαi2. YFP served as a negative control and ELMO1-YFP was a positive control. ( d ) CXCL12-induced ELMO1 colocalization with Gαi2 on the plasma membrane by confocal microscopy analysis. After stimulation with 100 ng ml −1 CXCL12 for 1 h at 37 °C, cells were fixed, permeabilized and blocked in 3% BSA. MDA-MB-231 cells were stained with anti-ELMO1, anti-Gαi2 antibodies and probed with an Alexa Fluor 488-conjugated or 546-conjugated secondary antibody. Colocalization efficiency was calculated through Image J software. ( e ) Knockdown of Gαi2 impaired CXCL12-induced membrane translocation of ELMO1. After stimulation with 100 ng ml −1 CXCL12 for 1 h at 37 °C, cells were fixed, permeabilized and blocked in 3% BSA. Twenty-five images were analysed by ImageJ software. Western blotting analysis of biochemical fractionation showed a clear enrichment of ELMO1 upon CXCL12 stimulation. Full size image Table 1 Mass spectrometry analysis. Full size table To identify the region of ELMO1 (727 aa) that interacted with Gαi2, we fused YFP to three fragments (FR1 1–300 aa, FR2 301–500 aa and FR3 501–727 aa) of ELMO1 and expressed each of them in MDA-MB-231 cells ( Fig. 2d ). Coimmunoprecipitation results showed that the ELMO1-YFP_FR1 but not ELMO1-YFP_FR2 or ELMO1-YFP_FR3, associated with Gαi2 ( Fig. 2c ), indicating that the N-terminal region of ELMO1 was involved in the interaction with Gαi2. These results indicate that CXCL12 stimulation promotes the interaction between Gαi2 and the N terminus of ELMO1, and the Gαi2-ELMO1/Dock180 pathway may have a role in chemokine receptor-mediated migration of the breast cancer cells. CXCL12 induces ELMO1 membrane translocation We next examined subcellular localization of Gαi2 and ELMO1, using an immunostaining analysis ( Fig. 2d and Supplementary Fig. S3A ). Before stimulation, fluorescent signals of Gαi2 but not those of ELMO1 were clearly detected on the plasma membrane. Upon CXCL12 stimulation, fluorescent signals of ELMO1 were clearly increased on plasma membrane, while those of Gαi2 remained unchanged. Using a pixel-by-pixel colocalization analysis, we found a strong colocalization of Gαi2 and ELMO1 on plasma membrane when the cells were stimulated with CXCL12 ( Fig. 2d and Supplementary Fig. S3A ). In addition, CXCL12 stimulation did not induce ELMO1 membrane translocation in the Gαi2 knockdown cells ( Fig. 2e and Supplementary Fig. S3B ). Biochemical fractionation analyses confirmed that CXCL12 stimulation induced an enrichment of ELMO1 in the membrane fraction, and this membrane enrichment of ELMO1 was not detected in Gαi2 knockdown cells ( Fig. 2e ). These results indicated that activation of CXCR4 chemokine receptor induced a Gαi2-dependent membrane translocation of ELMO1. CXCL12 induces membrane translocation and activation of Rac Chemokine GPCR has been shown to promote actin polymerization by activating the small G-proteins Rac1 and Rac2 (ref. 11 ). We therefore examined whether ELMO1 regulated the functions of Rac1 and Rac2 in breast cancer cells. Using an immunoprecipitation assay ( Fig. 3a ), we found that Rac1 and Rac2 associated with ELMO1-YFP, but not with the YFP control. In addition, CXCL12 and GTPγS stimulation, which activates Gαi signalling, promoted the association of both Rac1 and Rac2 with ELMO1-YFP, whereas PTX treatment, which blocks Gαi signalling, inhibited these associations ( Fig. 3a ). Using a biochemical fractionation analysis ( Fig. 3b ), we found that CXCL12 simulation resulted enrichment of Rac1 and Rac2 in the membrane fraction and that this membrane enrichment did not occur in ELMO1 knockdown (siELMO1) cells. Using confocal fluorescence microscopy, we confirmed that CXCL12-induced membrane translocation of Rac1 and Rac2, and that these translocations were suppressed in siELMO1 cells ( Fig. 3b and Supplementary Fig. S4 ). We then examined the role of ELMO1 in CXCL12-induced activation of Rac1 and Rac2 using a Rac activation assay ( Fig. 3c ). We found that CXCL12 stimulation induced activation of both Rac1 and Rac2, and that these activations were impaired when Gαi signalling was blocked by PTX or when ELMO1 was knocked down (siELMO1; Fig. 3c ). Together, these results suggest that CXCL12 activates a pathway in which activated Gαi2 and its association with the ELMO1/Dock180 complex promotes the membrane translocation and activation of Rac1 and Rac2 in breast cancer cells. 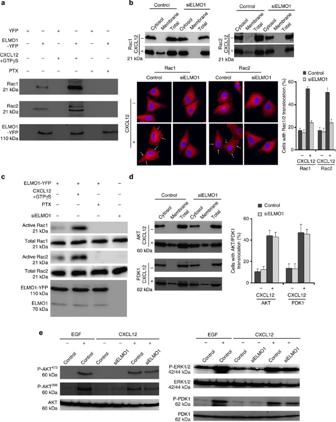Figure 3: CXCL12 induces membrane translocation and activation of Rac. (a) Coimmunoprecipitation assay of ELMO1-YFP, Rac1 and Rac2. The immunoprecipitation was performed by using the μMACS GFP isolation kit. The eluted proteins were separated by SDS–PAGE and probed with antibodies. (b) Knockdown of ELMO1 impaired CXCL12-induced membrane translocation of Rac1/2. After stimulation with 100 ng ml−1CXCL12 for 1 h at 37 °C, cells were fixed, permeabilized and blocked in 3% BSA. Twenty-five images were analysed by Image J software. Western blotting of biochemical fractionation showed that a clear enrichment of Rac1/2 upon CXCL12 stimulation and knockdown ELMO1 impaired CXCL12-induced Rac1/2 translocation. (c) Overexpression of ELMO1-YFP pulled down activated Rac1 and Rac2. Rac activation assay was performed by Rac Activation Assay Biochem Kit (Cytoskeleton, Inc.). Cleared lysates were obtained by centrifugation and incubated with PAK–PBD beads with rotation at 4 °C for 1 h. (d) siELMO1 had no effect in membrane translocation of AKT and PDK1. Western blotting showed a clear enrichment of AKT and PDK1 upon CXCL12 stimulation, and knockdown ELMO1 did not impair CXCL12-induced AKT and PDK1 translocation. (e) Western blotting analysis of phosphorylation of AKT308 or 473, ERK1/2 and PDK1. Control/MDA-MB-231 cells were stimulated by 10 ng ml−1EGF or 100 ng ml−1CXCL12 for 1 h. siELMO1/MDA-MB-231 cells were stimulated by 100 ng ml−1CXCL12 for 1 h. Total AKT, ERK1/2 and PDK1 served as control. Figure 3: CXCL12 induces membrane translocation and activation of Rac. ( a ) Coimmunoprecipitation assay of ELMO1-YFP, Rac1 and Rac2. The immunoprecipitation was performed by using the μMACS GFP isolation kit. The eluted proteins were separated by SDS–PAGE and probed with antibodies. ( b ) Knockdown of ELMO1 impaired CXCL12-induced membrane translocation of Rac1/2. After stimulation with 100 ng ml −1 CXCL12 for 1 h at 37 °C, cells were fixed, permeabilized and blocked in 3% BSA. Twenty-five images were analysed by Image J software. Western blotting of biochemical fractionation showed that a clear enrichment of Rac1/2 upon CXCL12 stimulation and knockdown ELMO1 impaired CXCL12-induced Rac1/2 translocation. ( c ) Overexpression of ELMO1-YFP pulled down activated Rac1 and Rac2. Rac activation assay was performed by Rac Activation Assay Biochem Kit (Cytoskeleton, Inc.). Cleared lysates were obtained by centrifugation and incubated with PAK–PBD beads with rotation at 4 °C for 1 h. ( d ) siELMO1 had no effect in membrane translocation of AKT and PDK1. Western blotting showed a clear enrichment of AKT and PDK1 upon CXCL12 stimulation, and knockdown ELMO1 did not impair CXCL12-induced AKT and PDK1 translocation. ( e ) Western blotting analysis of phosphorylation of AKT 308 or 473 , ERK1/2 and PDK1. Control/MDA-MB-231 cells were stimulated by 10 ng ml −1 EGF or 100 ng ml −1 CXCL12 for 1 h. siELMO1/MDA-MB-231 cells were stimulated by 100 ng ml −1 CXCL12 for 1 h. Total AKT, ERK1/2 and PDK1 served as control. Full size image ELMO1 is not required for PDK1/AKT and ERK1/2 activation CXCL12 binding to CXCR4 induces dissociation of heterotrimeric G-proteins into Gαi and Gβγ subunits, which regulate multiple pathways, including the activation of PDK1/AKT and ERK1/2 in breast cancer cells [24] , [25] , [26] . We found that ELMO1 was not essential for CXCL12-controlled pathways that activated PDK1/AKT or ERK1/2. Using a biochemical fractionation assay ( Fig. 3d ), we observed that CXCL12-induced membrane enrichment of PDK1 and AKT occurred in both control (MDA-MB-231) and ELMO1 knockdown (siELMO1) cells ( Fig. 3d and Supplementary Fig. S5 ). Furthermore, both CXCL12 and EGF induced a robust phosphorylation of PDK1 and AKT in siELMO1 cells at a level similar to that in parental control (MDA-MB-231) cells ( Fig. 3e ). In addition, CXCL12 stimulation induced clear ERK1/2 activation in both MDA-MB-231 (control) and knockdown of ELMO1 (siELMO1; Fig. 3e ). Thus, our results indicated that ELMO1 was not essential for the either PDK1/AKT or ERK1/2 activation pathways. ELMO2 has a role in breast cancer chemotactic responses ELMO2 shares 76% identity in amino acid sequence with ELMO1 and is also expressed in breast cancer cells ( Fig. 1a ), and thus, we investigated the role of ELMO2 in chemotaxis of MDA-MB-231 cells ( Fig. 4 ). As shown in Fig. 4a , ELMO2-YFP pulled down Dock180, Gαi2, Rac1 and Rac2. Moreover, although CXCL12 stimulation induced activation of both Rac1 and Rac2, it failed to do so when Gαi signalling was blocked by PTX or when ELMO2 was knocked down (siELMO2; Fig. 4b ). CXCL12-triggered actin polymerization and chemotaxis were also reduced in ELMO2 knockdown (siELMO2) cells ( Fig. 4c and d ). Our results suggest that ELMO1 and ELMO2 have similar roles in CXCL12-mediated signal transduction, leading to chemotaxis in MDA-MB-231 cells. Our observations that knockdown of either ELMO1 or ELMO2 in the cells results in defective chemotactic responses suggest that sufficient levels of ELMO1 and/or ELMO2 are required for robust CXCL12-triggered chemotaxis of the breast cancer cells. Consistent with this notion, we found that knockdown of both ELMO1 and ELMO2 further inhibited chemotaxis ( Fig. 4d ). In addition, expressing ELMO1-YFP in siELMO1 cells ( Supplementary Fig. S6A ), ELMO2-YFP in siELMO2 cells ( Fig. 4e ) or ELMO2-YFP in siELMO1 cells ( Fig. 4e ) could partially rescue chemotaxis defects in these cells. 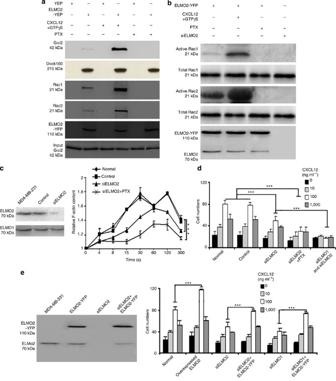Figure 4: ELMO2 has a role in breast cancer chemotactic responses. (a) Coimmunoprecipitation assay of ELMO2-YFP, Gαi2, Dock180, Rac1 and Rac2. The immunoprecipitation was performed by using the μMACS GFP isolation kit. The eluted proteins were separated by SDS–PAGE and probed with antibodies. Input Gαi2 was used as control. (b) Overexpression of ELMO2-YFP activated Rac1 and Rac2. Rac activation assay was performed by Rac Activation Assay Biochem Kit. Cleared lysates were obtained by centrifugation and incubated with PAK–PBD beads with rotation at 4 °C for 1 h. (c) Actin polymerization in siELMO2 cells was decreased. The value was measured at 0, 4, 8, 15, 30, 60, 120 and 300 s (points=mean of three independent experiments; scale bars=s.e.m.;n=6; two-way analysis of variance (ANOVA), ***P<0.0001). (d) Reduction of ELMO2 also inhibited chemotaxis of MDA-MB-231 cells, especially, when ELMO1 and ELMO2 were knocked down together (points=mean of three independent experiments; scale bars=s.e.m.;n=6; two-way ANOVA, ***P<0.0001). (e) Western blotting analysis: lane 1 was loaded with MDA-MB-231 cells, lane 2 with ELMO2-YFP/MDA-MB-231 cells, lane 3 with siELMO2/MDA-MB-231 cells and lane 4 with siELMO2+ELMO2-YFP (expressing ELMO2-YFP in siELMO2 cells). Overexpression of ELMO2 promoted chemotaxis (points=mean of three independent experiments; scale bars=s.e.m.;n=6; two-way ANOVA, ***P<0.0001), and overexpression of ELMO2 rescued the defects of siELMO1 (points=mean of three independent experiments; scale bars=s.e.m.;n=6; two-way ANOVA, ***P<0.0001) and siELMO2 cells (points=mean of three independent experiments; scale bars=s.e.m.;n=6; two-way ANOVA, ***P<0.0001). Figure 4: ELMO2 has a role in breast cancer chemotactic responses. ( a ) Coimmunoprecipitation assay of ELMO2-YFP, Gαi2, Dock180, Rac1 and Rac2. The immunoprecipitation was performed by using the μMACS GFP isolation kit. The eluted proteins were separated by SDS–PAGE and probed with antibodies. Input Gαi2 was used as control. ( b ) Overexpression of ELMO2-YFP activated Rac1 and Rac2. Rac activation assay was performed by Rac Activation Assay Biochem Kit. Cleared lysates were obtained by centrifugation and incubated with PAK–PBD beads with rotation at 4 °C for 1 h. ( c ) Actin polymerization in siELMO2 cells was decreased. The value was measured at 0, 4, 8, 15, 30, 60, 120 and 300 s (points=mean of three independent experiments; scale bars=s.e.m. ; n =6; two-way analysis of variance (ANOVA), *** P <0.0001). ( d ) Reduction of ELMO2 also inhibited chemotaxis of MDA-MB-231 cells, especially, when ELMO1 and ELMO2 were knocked down together (points=mean of three independent experiments; scale bars=s.e.m. ; n =6; two-way ANOVA, *** P <0.0001). ( e ) Western blotting analysis: lane 1 was loaded with MDA-MB-231 cells, lane 2 with ELMO2-YFP/MDA-MB-231 cells, lane 3 with siELMO2/MDA-MB-231 cells and lane 4 with siELMO2+ELMO2-YFP (expressing ELMO2-YFP in siELMO2 cells). Overexpression of ELMO2 promoted chemotaxis (points=mean of three independent experiments; scale bars=s.e.m. ; n =6; two-way ANOVA, *** P <0.0001), and overexpression of ELMO2 rescued the defects of siELMO1 (points=mean of three independent experiments; scale bars=s.e.m. ; n =6; two-way ANOVA, *** P <0.0001) and siELMO2 cells (points=mean of three independent experiments; scale bars=s.e.m. ; n =6; two-way ANOVA, *** P <0.0001). Full size image ELMO1 has a role in breast cancer metastasis in vivo To evaluate any potential contribution of ELMO proteins to the metastasis of breast cancer in vivo , we first examined the expression of ELMO1 and ELMO2 in tissue specimens from 81 patients with human invasive ductal carcinoma, which accounts for the majority of breast cancer cases, and 7 healthy controls using an immunohistochemical analysis. Positive ELMO1 staining was detected in 57 patient samples but only in 1 healthy control ( Fig. 5a , Table 2 and Supplementary Fig. S7A ). The expression of ELMO2 was also found to be higher in tumour tissues than in the normal breast tissues from healthy individuals ( Fig. 5b , Table 2 and Supplementary Fig. S7B ), suggesting that expression of ELMO1 and/or ELMO2 was elevated during tumorigenesis of breast cancer. Furthermore, analyses of lymph nodes from breast cancer patients revealed that 45 out of 51 lymph nodes with metastases stained positive for ELMO1, whereas only 12 out of 30 lymph nodes without metastases stained positive ( P =0.0001, χ 2 -statistics, Table 3 ). Moreover, ELMO1 expression was detected in 23 out of 26 distant metastasis cases (lung and liver with cancer cells), and in 34 out of 55 non-distance metastasis cases (lung and liver with no detectable cancer cells; Table 3 ). These results suggested that expressions of ELMO1 and/or ELMO2 were closely correlated with metastasis of breast cancers, either as a cause or as a consequence. 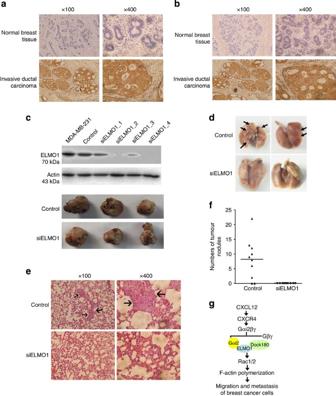Figure 5: ELMO1 has a role in breast cancer metastasisin vivo. (a) Immunohistochemical analysis of ELMO1 expression in invasive ductal breast carcinoma tissues and normal breast tissues. The entire sample (81 invasive ductal breast carcinoma tissues and 7 normal breast tissues) was blocked for 1 h. The antibodies and the dilution factors were as follows: ELMO1 (1:100), Polink-2 plus Polymer HRP Detection System for Goat Primary Antibody. (b) Immunohistochemical analysis of ELMO2 expression in invasive ductal carcinoma tissues and normal breast tissues. The entire sample (81 invasive ductal breast carcinoma tissues and 7 normal breast tissues) was blocked for 1 h. The antibodies and the dilution factors were as follows: ELMO2 (1:50), Polink-2 plus Polymer HRP Detection System for Goat Primary Antibody. (c) Western blotting analysis for four stable siELMO1 clones and comparison of tumour size in SCID mice. (d) Comparison of spontaneous lung metastasis and images of representative lung metastasis. (e) Human tumour foci on mouse lungs were visualized by haematoxylin and eosin staining. (f) The number of lung metastases was counted and plotted (n=10). (g) A model for ELMO1 regulated the migration and chemotaxis of breast cancer cells by associating with Dock180, Gαi2, Rac1 and Rac2. Figure 5: ELMO1 has a role in breast cancer metastasis in vivo. ( a ) Immunohistochemical analysis of ELMO1 expression in invasive ductal breast carcinoma tissues and normal breast tissues. The entire sample (81 invasive ductal breast carcinoma tissues and 7 normal breast tissues) was blocked for 1 h. The antibodies and the dilution factors were as follows: ELMO1 (1:100), Polink-2 plus Polymer HRP Detection System for Goat Primary Antibody. ( b ) Immunohistochemical analysis of ELMO2 expression in invasive ductal carcinoma tissues and normal breast tissues. The entire sample (81 invasive ductal breast carcinoma tissues and 7 normal breast tissues) was blocked for 1 h. The antibodies and the dilution factors were as follows: ELMO2 (1:50), Polink-2 plus Polymer HRP Detection System for Goat Primary Antibody. ( c ) Western blotting analysis for four stable siELMO1 clones and comparison of tumour size in SCID mice. ( d ) Comparison of spontaneous lung metastasis and images of representative lung metastasis. ( e ) Human tumour foci on mouse lungs were visualized by haematoxylin and eosin staining. ( f ) The number of lung metastases was counted and plotted ( n =10). ( g ) A model for ELMO1 regulated the migration and chemotaxis of breast cancer cells by associating with Dock180, Gαi2, Rac1 and Rac2. Full size image Table 2 ELMO1/2 expression in breast tissue. Full size table Table 3 Correlation of ELMO1 expression with clinical pathologic parameters and other biomarkers. Full size table We then evaluated the in vivo contribution of ELMO1 to metastasis of breast cancer cells, using an experimental mouse model for metastasis of breast cancer [1] . As both ELMO1 and ELMO2 were needed for robust chemotaxis, knockdown of one isoform, ELMO1, should be sufficient to inhibit cancer cell metastasis. Clone 2 and clone 4 of siELMO1 cells were mixed and injected into the mammary fat pad of severe combined immune deficient (SCID) mice, and siRNA cells were used as a control. Six weeks after the injections, the sizes of primary tumours were found to be similar in mice that were injected with siELMO1 cells or siRNA cells (control; Fig. 5c ), indicating that ELMO1 was not essential for tumour growth in vivo . To evaluate metastasis of the breast cancer cells, we examined tumour formation in the lung, a secondary organ of the breast cancer metastasis ( Fig. 5d ). Tumour foci were clearly formed in the lungs of mice injected with siRNA cells (control). In contrast, no foci were detected in the lungs of mice injected with siELMO1 cells ( Fig. 5d ). We further examined tumour cells in lungs using a histochemical staining with haematoxylin and eosin ( Fig. 5e and Supplementary Fig. S7C ). Although extensive tumour foci were found in eight out of ten mice that were injected with siRNA cells (control), no tumour foci were detected in the lungs of the mice injected with siELMO cells ( Fig. 5f ). Thus, our results demonstrate that although not essential for tumour growth in its original site, ELMO1 is clearly required for the metastasis of human breast cancer in vivo . In this study, we have identified a chemokine receptor-controlled pathway, consisting of Gαi2, the ELMO1/Dock180 complex, Rac1 and Rac2, which activates actin polymerization in human breast cancer cells ( Fig. 5g ). We show that CXCL12 stimulation regulates the ELMO1/Dock180 function via promoting the association between Gαi2 and ELMO1 in the breast cancer cells. Our results of the pull-down/mass spectrometry and coimmunoprecipitation analyses indicate that Gαi2 associates with ELMO1, which forms a stable complex with Dock180. Gαi2 interacts with the N-terminal portion of ELMO1. This interaction is promoted by CXCL12 stimulation and inhibited by blocking Gi signalling (PTX treatment), whereas the association between ELMO1 and Dock180 is independent of CXCL12 stimulation or Gi signalling. Furthermore, CXCL12 stimulation induces a membrane translocation of ELMO1, which depends on Gαi2. Our results suggest that ELMO1 has a critical role in the activation of Rac1 and Rac2 in breast cancer cells. CXCL12 stimulation induces membrane translocation and activation of Rac1 and Rac2, and these activities require both Gi signalling and ELMO1. Together, our data suggest that binding of CXCL12 to its receptor activates the Gαi2 subunit, upon which it associates with the ELMO1/Dock180 complex, translocates from cytosol to membrane, to activate Rac1 and Rac2, and thereby promote actin polymerization in the breast cancer cells. Breast cancer cells express both ELMO1 and ELMO2, but not ELMO3. Both ELMO1 and ELMO2 appear to have a similar role in mediating chemotaxis of breast cancer cells. Upon stimulation by CXCL12, both ELMO1 and ELMO2 interact with Gαi2 and activate Rac1 and Rac2. Knockdown of either ELMO1 or ELMO2 impairs actin polymerization. Overexpression of either ELMO1 or ELMO2 rescues the migration defects of siELMO1 cells. Thus, functions of ELMO1 and ELMO2 appear to be interchangeable. There are three Gαi (Gαi1, Gαi2 and Gαi3) in breast cancer cells. Our mass spectrometry analysis has only revealed Gαi2 as being associated with ELMO1. Knockdown of Gαi2 inhibits CXCL12-induced ELMO1 translocation, suggesting that the function of Gαi2 is irreplaceable. The roles of Gαi1 and Gαi3 in chemotaxis of breast cancer cells need further investigation. We have shown that the ELMO1 pathway is critical for CXCL12-mediated migration and invasion of the breast cancer cells in vitro and metastasis of breast cancer in vivo . Blocking Gi signalling by PTX or knocking down ELMO1 inhibits CXCL12-triggered actin polymerization, and CXCL12-mediated chemotaxis and invasion of breast cancer cells in vitro . In vivo , ELMO1 is expressed at a relatively high level in human breast cancer samples, and the expression correlates with lymph node metastasis and distant metastasis in breast cancer patient samples. Furthermore, downregulating ELMO1 in breast cancer cells negatively affects tumour formation in the lung, suggesting that ELMO1 is required for breast cancer cell migration from the original site to a secondary organ in the mouse model. The EGF and its receptor (a tyrosine kinase receptor) control several signalling pathways that have been implicated in promotion of tumour progression, invasion and metastasis in various cancers including breast cancers [24] , [27] , [28] . PDK1/AKT or ERK1/2 can be activated by either EGF receptor or CXCR4 GPCR in the breast cancer cells ( Fig. 3e ). Previous studies have shown that the PDK1/AKT pathways and the ERK/MAPK pathways have critical roles in the growth and the migration of breast cancers [24] , [29] . The EGF receptor also regulates a pathway, consisting of PLC, PIP3 and cofilin, to promote actin polymerization for invasion and metastasis of breast cancer cells [30] . Interestingly, neither ELMO1 nor ELMO2 is required for either CXCL12- or EGF-induced activation of PDK1/AKT or ERK1/2 ( Fig. 3e and Supplementary Fig. S9A ), or for EGF-induced migration of the breast cancer cells in vitro ( Supplementary Fig. S1B ). However, both ELMO1 and ELMO2 are required for CXCL12-induced cell migration and metastasis in vivo . It appears that multiple extracellular cues and the pathways they control are working together in the breast cancer cells for directing migration and invasion during metastasis of breast cancer in vivo . Future studies are needed to understand how these pathways work together to control metastasis of breast cancer. It is worth noting that ELMO1 has been identified as a modifier of breast cancer risk for BRCA mutation carriers [31] , suggesting a role of ELMO1 in human breast cancer patients. It would be useful to establish the value of other signalling components in these pathways, such as ELMO1, as biomarkers for the diagnosis and treatment of breast cancer metastasis. Cell culture and reagents MDA-MB-231 cells (American Type Culture Collection); HEK293T, T47D and MCF-7 cells (American Type Culture Collection); Lipofectamine 2000 (Invitrogen); ELMO1-YFP and ELMO2-YFP construction (GeneCopoeia); SilverQuest Staining Kit (Invitrogen); CXCL12 (R&D Systems, Inc.); RPMI-1640 medium and FBS from Hyclone; Alexa Fluor 568-phalloidin, Alexa Fluor 488-conjugated donkey anti-goat IgG, Alexa Fluor 546-conjugated goat anti-mouse IgG and Alexa Fluor 546-conjugated goat anti-rabbit IgG (Molecular Probes, Inc.); anti-GFP antibody (Roche); anti-ELMO1, anti-ELMO2, anti-ELMO3 and anti-PDK1 antibody from Abcam Inc.; anti-Dock180, anti-AKT, anti-Phospho-AKT 473or308 , anti-ERK1/2, anti-Phospho-ERK1/2 and anti-Phospho-PDK1 from Cell Signaling Technology; anti-Rac1 (BD Biosciences); anti-Rac2 and anti-Gαi2 antibody (Santa Cruz Biotechnology, Inc.); anti-mouse, rabbit and goat secondary antibody (Jackson Immuno Research Laboratories, Inc.); μMACS Epitope Tag Protein Isolation Kit (Miltenyi Biotec, Inc.); ON-TARGETplus SMARTpool, si-human ELMO1 and ON-TARGETplus Non-targeting siRNA#1 (Dharmacon, Inc.); Matrigel Invasion Chambers (BD Biosciences); Rac Activation Assay Biochem Kit (Cytoskeleton, Inc.); Pertussis Toxin (Calbiochem); ELMO1 siRNA, ELMO2 siRNA, Gαi2 siRNA (Shanghai GeneChem Co., Ltd); Polink-2 plus Polymer HRP Detection System For Goat Primary Antibody (ZSGB-BIO Co., Ltd); SCID mice from Wei Tong Li Hua Experimental Animal Co. Ltd. siRNA and transfection Cells were plated in a six-well plate for 24 h before transfection. Transfection was done with Lipofectamine 2000 according to the manufacturer’s instructions using ON-TARGETplus SMARTpool human ELMO1 and ON-TARGETplus Non-targeting siRNA#1 as control. The target sequences of ON-TARGETplus SMARTpool human ELMO1 were 5′-UGACAAGCAUGAGUACUGU-3′, 5′-GCAUUACGGAGACUUAGAA-3′, 5′-GAACUCGCUUUCUCCAUCU-3′ and 5′-GGACUGCCCUCAUAUGAAA-3′. Sequences of ELMO2 siRNA were 5′-ACUGAGGAGGAUUGCAUUUTT-3′, 5′-GAUGGCCCAUCAGCUAUAUTT-3′ and 5′-AGCAUCUCCGGUCUAUAAUTT-3′. Sequence of the non-silencing control was 5′-UUCUCCGAACGUGUCACGUTT-3′. Sequence of Gαi2 siRNA: 5′-CCGATGTCATCATCAAGAA-3′, 5′-AGAGTAAGTTTGAGGACCT-3′ and 5′-TATTCGATAGCATCTGCAA-3′, with 5′-UUCUCCGAACGUGUCACGUTT-3′ as the non-silencing control. For the knockdown of ELMO2 and Gαi2, the methods were the same. For plasmid transfection, cells were plated in a 10-cm dish for 24 h before transfection. Identification of proteins that interact with ELMO1/ELMO2 Cells expressing ELMO1-YFP, ELMO2-YFP or YFP (as the control) were stimulated by 100 ng ml −1 CXCL12. The immunoprecipitation was performed by using the μMACS GFP isolation kit according to the manufacturer’s protocol. Briefly, lysates were obtained by centrifugation at 10,000 g for 10 min at 4 °C. The lysates were incubated with μMACS anti-GFP MicroBeads on ice for 30 min. Proteins were eluted with elution buffer after properly washing the microbeads. Protein identification work was carried out at ProtTech, Inc. (Norristown, PA, USA). Coimmunoprecipitation MDA-MB-231 cells expressed ELMO1-YFP, ELMO2-YFP or its fragments. The immunoprecipitation was performed by using the μMACS GFP isolation kit. Proteins were eluted with elution buffer. The eluted proteins were separated by SDS–PAGE and probed with anti-Gαi2, anti-Dock180, anti-Rac1 or two antibodies. MDA-MB-231 cells expressing YFP were used as a negative control. Isolation of membrane fractions Cells on 10-cm plates were lysed by using 500 μl of buffer per plate. The lysate was transferred into a 1.5-ml Eppendorf tube, passed through a 25-G needle ten times using a 1-ml syringe, and kept on ice for 20 min before centrifuging at 720 g at 4 °C for 5 min to pellet down the nucleus. The supernatant was transferred into a fresh tube and centrifuged at 10,000 g at 4 °C for 10 min. The supernatant (containing cytosolic and membrane fractions) was subsequently centrifuged at 100,000 g at 4 °C for 60 min to separate the cytosolic (supernatant) and the membrane (pellet) fractions. The pellet was resuspended in 400 μl of the fractionation buffer (250 mM sucrose, 20 mM HEPES, 10 mM KCl, 1.5 mM MgCl 2 , 1 mM EDTA, 1 mM EGTA, 1 mM dithiothreitol and proteinase inhibitor cocktail) and centrifuged at 100,000 g at 4 °C for 45 min. The membrane pellet was dissolved in SDS–PAGE lysis buffer with 10% glycerol and 0.1% SDS, and kept at −20 °C until use. Rac activation assay The Rac activation assay was performed by affinity precipitation following the protocol in the Rac Activation Assay Biochem Kit. Briefly, MDA-MB-231 cells expressing YFP (control), ELMO1-YFP or ELMO2-YFP were treated with either CXCL12 alone, CXCL12 and GTPγS combined or PTX alone, before being solubilized with lysis buffer containing protease inhibitors. Lysates were cleared by centrifugation at 10,000 g at 4 °C for 2 min and then incubated with PAK–PBD beads with rotation at 4 °C for 1 h. Subsequently, proteins bound to the beads were dissociated with SDS–PAGE sample buffer, separated by SDS–PAGE and analysed for Rac1 or Rac2 by western blotting. Scratch assay Control and ELMO1 siRNA cells were plated in six-well plates and formed a fluent monolayer. The medium was replaced by a RPMI medium supplied with 1% bovine serum albumin (BSA). One of ELMO1 siRNA wells was pretreated with 0.1 μg ml −1 PTX in medium for 2 h. Then they were lined out with an even trace in the middle using a 10-μl pipette tip. The distance of the wounds was measured within an appropriate time (0, 3, 6, 9, 12 and 24 h) under a light microscope ( × 100). In vitro transwell assay In vitro transwell assays were performed as described by Sun et al . [28] Briefly, CXCL12 (0, 10, 100 and 1,000 ng ml −1 ) was loaded into the lower chambers and the cell suspension (5 × 10 5 cells per ml) in binding medium (RPMI-1640, 0.1% BSA and 25 mM HEPES) was then loaded into the upper chambers. The chambers were incubated in 5% CO 2 at 37 °C for 3 h. Then the filter membrane was washed, fixed and stained. The number of migrating cells was counted in three separate fields ( × 400) by light microscopy. MTT assay Briefly, cells were plated in 96-well plates. Twenty microlitres of the stock MTT solution (5 mg ml −1 ) in PBS were added to each well at different time and incubated for 4 h at 37 °C. Cell viability was calculated by the absorbance at 570 nm. Matrigel invasion assay The invasion of cells in vitro was measured by the invasion of cells through Matrigel-coated transwell chambers. Cell suspension was prepared (5 × 10 5 cells per ml) in binding medium. CXCL12 (100 ng ml −1 ) was added to the lower well. After 24 h of incubation (37 °C, 5% CO 2 ), the invading cells were fixed and stained. The number of invading cells was counted under a microscope in six predetermined fields (total magnification, × 400). F-actin polymerization assay Cellular F-actin measurement was done as described by Tsuboi [32] . Briefly, after addition of 100 ng ml −1 CXCL12, cells were incubated for the indicated time point at 37 °C. Cells were then fixed by 4% paraformaldehyde for 5 min and permeabilized by 0.1% Triton X-100 for 10 min. The cells were incubated with Alexa Fluor 568-phalloidin for 6 min. F-actin content was measured by a microplate fluorescence reader with an excitation wavelength of 578 nm and an emission wavelength of 600 nm. Results were expressed as relative F-actin content, where F-actin t/F-actin 0=(fluorescence t/mg ml −1 )/(fluorescence t0/mg ml −1 ). Immunofluorescence confocal microscopy Briefly, cells were plated in 12-well plates containing sterile coverslips, allowed for 24 h growth, and starved in serum-free RPMI-1640 for 3 h. After stimulation with 100 ng ml −1 CXCL12 for 1 h at 37 °C, the cells were fixed with 4% paraformaldehyde, permeabilized in 0.1% Triton X-100 in PBS and blocked in 3% BSA. Cells were stained with anti-ELMO1 and anti-Gαi2 antibodies, and probed with an Alexa Fluor 488-conjugated or 546-conjugated secondary antibody. Cells were stained with anti-ELMO1, Rac1, Rac2, PDK1 or AKT antibody, and probed with an Alexa Fluor 488-conjugated or 546-conjugated as the secondary antibody. Coverslips were mounted and visualized with confocal laser scanning microscopy (Olympus FV1000). Colocalization efficiency was calculated through ImageJ software (NIH, Bethesda, MD). Twenty-five images were analysed. Immunohistochemical assay Archival paraffin blocks of normal breast tissue and invasive breast cancer cases were obtained from the Department of Breast Cancer, Tianjin Medical University Cancer Institute and Hospital. Comprehensive staining intensity and the percentage of positive cells were considered as semiquantitative analysis by immunohistochemistry staining standard. Score for intensity of staining was defined as ‘0’=undetectable staining, ‘1’=yellow staining, ‘2’=brown staining and ‘3’=yellow–brown staining. Score for the positive percentage of cells was shown as follows: ‘0’, number of positive cells<10%; ‘1’, number of positive cells between 10 and 40%; ‘2’, number of positive cells between 40 and 70%; and ‘3’, number of positive cells≥70%. Sum of the above two score ‘0–2’ was considered negative; ‘3–6’ was considered positive. The entire sample (81 invasive ductal breast carcinoma tissues and 7 normal breast tissues) was blocked for 1 h. The antibodies and the dilution factors were as ELMO1 (1:100) and ELMO2 (1: 50), and Polink-2 plus Polymer HRP Detection System for Goat Primary Antibody was used for the detection. The results were analysed by χ 2 -statistics. In vivo spontaneous metastasis assay Metastasis assays were performed as described previously [24] . Briefly, siELMO1 and control cells were grown until the log phase, trypsinized and washed three times with serum-free medium. Four-week-old female SCID mice were injected subcutaneously into the mammary fat pads with 2 × 10 6 cells ( n =10 per group). After 6 weeks, the mice were killed. To examine spontaneous metastasis, the lungs were fixed with formalin and embedded in paraffin. Serial sections and haematoxylin and eosin staining were performed to detect lung micrometastasis. Additional information How to cite this article: Li, H. et al . Association between Gαi2 and ELMO1/Dock180 connects chemokine signalling with Rac activation and metastasis. Nat. Commun. 4:1706 doi: 10.1038/ncomms2680 (2013).